Iodine-catalyzed diazo activation to access radical reactivity Transition-metal-catalyzed diazo activation is a classical way to generate metal carbene, which are valuable intermediates in synthetic organic chemistry. An alternative iodine-catalyzed diazo activation is disclosed herein under either photo-initiated or thermal-initiated conditions, which represents an approach to enable carbene radical reactivity. This metal-free diazo activation strategy were successfully applied into olefin cyclopropanation and epoxidation, and applying this method to pyrrole synthesis under thermal-initiated conditions further demonstrates the unique reactivity using this method over typical metal-catalyzed conditions. Diazo compounds are versatile building blocks in chemical synthesis due to their ability to serve as carbene precursors under various metal-catalyzed conditions [1] , [2] , [3] , [4] , [5] , [6] . While typical metal carbenes are electrophilic, Zhang and other groups [7] , [8] , [9] reported a series of novel Co(II)-porphyrin carbene complexes with strong Co-C single-bond character, which displayed carbene carbon radical reactivity (Fig. 1a ). Mechanistic investigation and new transformations have been reported [10] , [11] , [12] , [13] , [14] , [15] , [16] , demonstrating the unique reactivity of these metal carbene radicals. Those seminal work disclosed the possibility of activating diazo compounds as radical precursors. However, as the general need in synthesis, new methodology is always highly desirable, especially those with significant different activation mode under distinct mechanism. Fig. 1 Catalytic diazo compound activation: carbene vs. radical. a Metal-catalyzed diazo compound activation. b This work: access diazo radical reactivity through simple iodine catalysis Full size image Herein, we report our discovery of iodine-catalyzed diazo activation and application of this method toward olefin cyclopropanation (Fig. 1b ). Importantly, this method revealed a metal-free catalytic system to access diazo radical reactivity under mild conditions. Moreover, the ability to tolerate challenging substrates such as enamides ensure the successful synthesis of substituted pyrroles through cyclopropanation and sequential rearrangement in one pot, which highlights the advantage of this methodology over the typical metal-catalyzed system. Combining iodine-catalyzed diazo activation and photocatalysis This iodine-catalyzed diazo activation originated from an accidental discovery [17] , [18] , [19] , [20] . It has been recently reported that aryl diazonium salts (ArN 2 + ) are effective oxidants in promoting gold(I) oxidation to gold(III) [21] , [22] , [23] . To extend the reactivity to alkyl diazonium salt, we hypothesized that treating diazo compound with proper electrophile could generate a reactive diazonium intermediate in situ, which might serve as a potential oxidant for gold(I) oxidation. To explore the feasibility of this idea, we investigated reactions of ethyl diazoacetate (EDA) 1a with various electrophiles. Interestingly, treating EDA 1a with I 2 led to the formation of ethyl diiodoacetate 1a′ in nearly quantitative yield even at room temperature, suggesting rapid decomposition of transient intermediate A (Fig. 2a ). Notably, Suero and coworkers [24] recently reported an interesting styrene cyclopropanation with CH 2 I 2 under photoredox conditions. As proposed by the author, the iodo-substituted methyl radical was formed via a photoredox reductive quenching cycle, which subsequently reacted with an alkene to form radical intermediate B . However, access reductants ( i -Pr 2 EtN and Na 2 S 2 O 3 ) are required to initiate the reductive Ru I /Ru II cycle and scavenge the resulting I 2 (Fig. 2b ). Fig. 2 Synthesis of diiodoacetate 1a′ and our hypothesis. a Rapid reaction between diazo 1a and I 2 . b Olefin cyclopropanation via photo-initiated CH 2 I 2 activation reported by Suero. c Our proposal: combining iodine promoted diazo activation and photo-initiation Full size image With the realization of diiodo compound 1a′ by reacting diazo compound with I 2 under mild conditions, we wondered whether this process could be combined with photo activation to access diazo radical reactivity. Notably, it has been reported that electron-deficient alkyl halides could serve as effective oxidants to convert [Ru(bpy) 3 ] 2+ into [Ru(bpy) 3 ] 3+ under photochemical conditions [25] , [26] , [27] , [28] , [29] . Thus, it is reasonable to expect 1a′ to serve as an oxidant and promote oxidative Ru II /Ru III cycle (Fig. 2c ). Addition of the resulting carbon radical C to alkene will form the radical intermediate B′ , which undergoes cyclization through the release of an iodine radical. The iodine radical would react with iodide to form anionic radical I 2 −• . Ultimately, [Ru(bpy) 3 ] 3+ acquires an electron from I 2 −• to regenerate I 2 and [Ru(bpy) 3 ] 2+ . Compared with the process reported by Suero and coworkers [24] , this proposed approach is more atom economic since only catalytic amount of iodine could initiate the radical process to avoid the usage of access reductants ( i -Pr 2 EtN and Na 2 S 2 O 3 ). 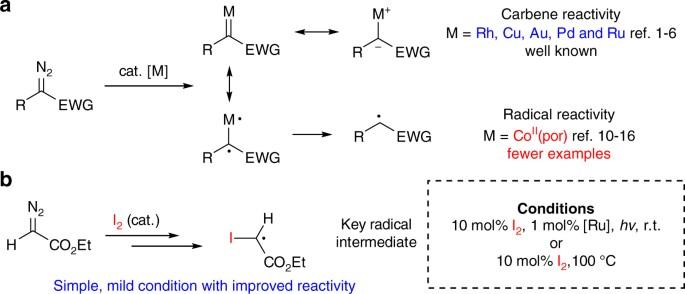Fig. 1 Catalytic diazo compound activation: carbene vs. radical.aMetal-catalyzed diazo compound activation.bThis work: access diazo radical reactivity through simple iodine catalysis Olefin cyclopropanation under photo-conditions To our delight, the desired cyclopropanation product 3a was obtained in 96% yield (dr = 1.9:1, diastereomeric ratio) using the combination of I 2 (10 mol%) and Ru(bpy) 3 Cl 2 (1 mol%) as catalysts (Table 1 ). Control experiments clearly demonstrated that iodine and photo catalysts were indispensable for this transformation. The reaction worked well with either blue or white light, while no product 3a was obtained if reacting in the dark, which is consistent with the proposed photo-initiated mechanism. Ir(dtbbpy)(bpy) 2 PF 6 could also catalyze this reaction with 65% yield, while organo-photosensitizer eosin Y could not promote this transformation. Diiodide compound 1a′ could substitute I 2 as an effective catalyst for this transformation, giving 3a in 94% yield. This result clearly supported our hypothesis that 1a′ is the key intermediate for photo-initiation. No 3a was observed when using Br 2 instead of I 2 as catalyst [30] , [31] , [32] . Interestingly, reaction of alkene and 1a′ under photo activation conditions (no diazo 1a and I 2 ) gave only trace amount of product. This is likely caused by the formation of large amount of I 2 (without the addition of extra reductants such as Na 2 S 2 O 3 ), which would quench the photo-excited state of the catalyst *[Ru(bpy) 3 ] 2+ and prevent photocatalytic cycle from happening [33] . Conducting the reaction ( 2a and 1a′ ) under Suero’s conditions (with i -Pr 2 EtN and Na 2 S 2 O 3 in MeCN) gave the desired product 3a in 35% yield [24] . These results highlighted the overall high efficiency of this photo-catalyzed Ru II /Ru III oxidative cycle by simply using diazoacetate and catalytic iodine. (2,2,6,6-Tetramethylpiperidin-1-yl)oxyl or (2,2,6,6-tetramethylpiperidin-1-yl)oxidanyl (TEMPO) could effectively quench the reaction, which was consistent with the proposed radical mechanism. Interestingly, when conducting the reaction with olefin 2b , <10% 2b conversion was observed with 10 mol% I 2 as catalyst. Analyzing the reaction mixture revealed the formation of diiodide compound 4 as the major product through radical-promoted cyclopropane ring opening. Increasing the amount of I 2 to 1 equiv. gave the desired diiodide product 4 in 75% isolated yield ( E / Z = 15:1) (Fig. 3 ). These results not only demonstrated formation of radical intermediates D and E in a typical radical clock experiment, but also revealed faster iodination of radical E over either hydrogen radical elimination or radical cyclization [34] . Table 1 Optimization of the reaction conditions under photo-initiated conditions Full size table Fig. 3 Radical clock experiment. Proposed mechanism for the synthesis of 4 Full size image With the optimized conditions revealed, we investigated the reaction scope under photo-initiated conditions. 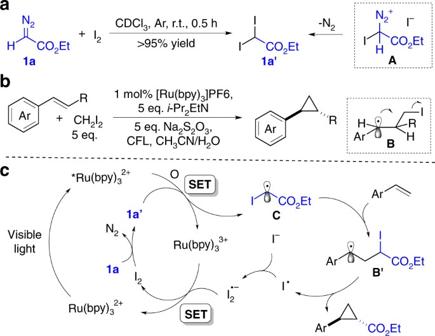Fig. 2 Synthesis of diiodoacetate1a′and our hypothesis.aRapid reaction between diazo1aand I2.bOlefin cyclopropanation via photo-initiated CH2I2activation reported by Suero.cOur proposal: combining iodine promoted diazo activation and photo-initiation The results are summarized in Table 2 . Styrenes bearing both electron-donating and electron-withdrawing groups are all suitable for this transformation, giving desired products ( 3a – 3h ) in good to excellent yields (around 2:1 dr ratio). Other arene-substituted olefins also works well ( 3i , 3k – 3m ). However, the reactions only gave diminished yields for highly electron-deficient alkenes, such as 2-vinylpyridine, chalcone, and p -NO 2 styrene. In addition, messy reactions were observed for diene, methyl 2-phenylacrylate, and vinyl ether substrates. Table 2 Reaction scope under photo-initiated conditions Full size table Iodine-catalyzed diazo activation toward olefin cyclopropanation under thermal conditions Although this iodine-catalyzed diazo activation under photo-initiation provided a simple and novel approach to access diazo radical reactivity, it only displayed a limited substrate scope. Control experiments disclosed two main reasons: (1) Ru(bpy) 3 Cl 2 would be quenched by certain alkenes, such as vinylferrocene, p -NO 2 -styrene and enamide; (2) some alkenes (vinyl ether and dienes) would decompose under photo-conditions (see details in Supplementary Figs. 2 and 3 ). To further expand this methodology to more challenging substrates such as photo-sensitive alkenes and electron-deficient alkenes, we wondered whether alternative ways to generate radical intermediate C is feasible. We hypothesized this could be achieved from C–I bond homo-dissociation of diiodide compound 1a′ at elevated temperatures. 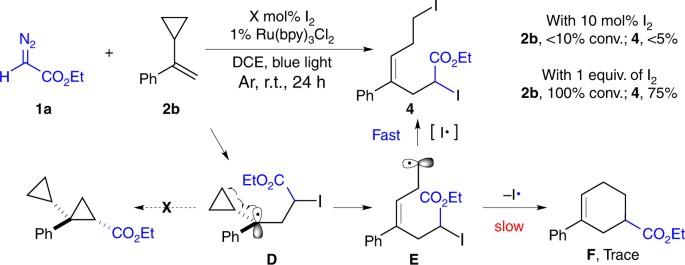Fig. 3 Radical clock experiment. Proposed mechanism for the synthesis of4 Unfortunately, heating reaction mixtures of 2a and 1a′ at 100 °C gave no conversion of alkene 2a after 24 h (Table 3 , entry 1), suggesting no formation of radical C [35] . The conversion of 2a was <10% while reacting with diazo 1a under simple heating conditions [36] . To our delight, adding 10 mol% I 2 into reaction mixtures of 2a and 1a at 100 °C successfully delivered the desired cyclopropane 3a in nearly quantitative yield (entry 3). Interestingly, increasing the amount of I 2 to 1 equiv. completely quenched the reaction (entry 4), suggesting the rapid formation of 1a′ when treating 1a with I 2 , which is not a valid substrate alone for this reaction as shown in entry 1. Furthermore, switching I 2 catalyst to 10 mol% 1a′ gave same excellent yield of 3a (entry 5). These results clearly demonstrated that reaction between diiodide compound 1a′ and diazo 1a at elevated temperature produced the active intermediate that promoted the overall transformation. In addition, only trace amount of product 3a was formed at 80 °C, and other catalysts (Br 2 , KI, NIS) were invalid for this transformation. Table 3 Optimization of the reaction conditions under thermal-initiation conditions Full size table To explore the reaction mechanism under the thermal conditions, several control experiments were performed as shown in Fig. 4 . First, similar to photo-initiated conditions, reaction was completely quenched by TEMPO and intermediate G was successfully detected by gas chromatography–mass spectrometry (Supplementary Fig. 1 ). Radical clock experiment give the desired diiodide product 4 with 80% yield ( E:Z = 4:1). Importantly, electron paramagnetic resonance (EPR) experiments were performed, and, fortunately, both nitrogen radical and carbon radical were clearly detected (see EPR spectra in Supplementary Fig. 4 ). Although the exact mechanism requires further investigation, based on current experimental results, it is reasonable to speculate the formation of active reaction intermediate upon mixing 1a and 1a′ (such as H ). This intermediate would generate nitrogen radical I and/or carbon radical C via single electron transfer (SET) process at elevated temperature. Ultimately, the cyclopropane was formed through intramolecular radical substitution as shown in Fig. 2 . Fig. 4 Evidences for radical process under thermal condition. a Radical trapping and radical clock experiments. b Proposed mechanism for the generation of intermediate C Full size image Encouraged by the simple and metal-free diazo activation method under thermal conditions, we explored the reaction scope, especially the challenging substrates that photo-initiated method failed to work. 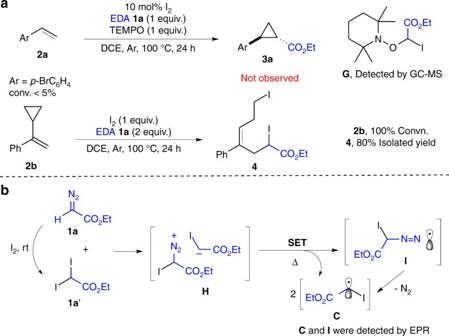Fig. 4 Evidences for radical process under thermal condition.aRadical trapping and radical clock experiments.bProposed mechanism for the generation of intermediateC The results are summarized in Table 4 . Compared with photo-initiated conditions, the thermal-initiation reactions were significantly cleaner, giving higher yields in almost all cases (i.e., 3j from 20 to 94%, 3l from 60 to 92%). Moreover, alkene substrates that are not suitable for photo-conditions, such as 1-nitro-4-vinylbenzene and vinylferrocene, worked well under the thermal conditions, giving the desired products 3p and 3t in 94% and 76% yields, respectively. Furthermore, vinyl ether ( 3u ), methyl 2-phenylacrylate ( 3v ), eneyne ( 3w ), and diene ( 3 s ) are all suitable for this new thermal condition, providing desired products in good yields. The conjugated diene and eneyne also gave excellent regio-selectivity. Other types of diazo compounds were also prepared and applied to this transformation. Interestingly, acceptor–acceptor-type diazo compound with a ketone substitution reacted with alkene and gave dihydrofuran 3× through a sequential cyclopropane rearrangement. On the other hand, the donor–-acceptor-type diazo compounds were inactive under this new condition likely due to the increased steric hindrance and competing carbene dimerization. Overall, this thermal approach for iodine-catalyzed diazo activation exhibits a very broad substrate scope. The fact that both electron-rich and electron-deficient alkenes works well under this condition is in sharp contrast with traditional metal carbenoid chemistry and more resembles the Co(II)–porphyrin-associated carbene radicals [8] . Table 4 Reaction scope under thermal-initiated conditions Full size table Iodine-catalyzed pyrrole synthesis from enamides and diazo compounds To further demonstrate the uniqueness of this iodine-catalyzed diazo activation method, we focused on transformations that are not suitable with typical metal-catalyzed diazo substrates. As shown in Fig. 5 , typical metal catalysts, such as Rh, Cu, Pd, and Au (see Supplementary Table 3 ), could not promote this cyclopropanation of enamide, giving low starting material conversion with EDA decomposition as the major products. To evaluate the new iodine-catalyzed diazo activation method, we investigated this challenging transformation. To our delight, pyrrole 6a was observed with 87% yield under thermal-initiation condition, while almost no reaction under photo-initiated conditions. Monitoring the reaction process revealed the formation of cyclopropane 6c′ , which would convert to 6c through cyclopropane ring opening. Compound 6c′ was isolated and charged under the thermal conditions, giving the desired pyrrole 6c in quantitative yield, which further confirmed the proposed reaction cascade. To the best of our knowledge, this is the first synthesis of pyrroles from enamides and diazo compounds. Fig. 5 Thermally initiated iodine-catalyzed pyrrole synthesis. 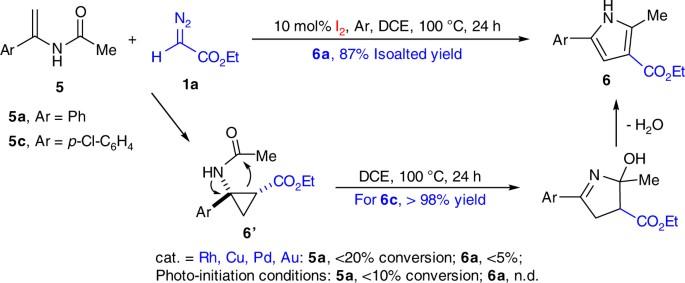Fig. 5 Thermally initiated iodine-catalyzed pyrrole synthesis. Generation pyrrole from the key cyclopropane intermediate6′ Generation pyrrole from the key cyclopropane intermediate 6′ Full size image The reaction scope of this new pyrrole synthesis is summarized in Table 5 . Similar to the cyclopropanation, various aryl and alkyl enamides are well suited for this transformation, giving the corresponding pyrroles in good yields ( 6a – 6o ). Notably, the highly sterically congested tetrasubstituted pyrroles could also be formed in moderate yield, indicating the remarkable efficiency of this new transformation ( 6p and 6q ). Other diazo esters and ketones were applied to this reaction and gave the desired products in good to excellent yields ( 6r – 6x ). To showcase the practicality of this methodology, a gram-scale reaction was performed, and 6a was obtained in 80% yield (1.83 g). Compared with previously reported metal-catalyzed formal [3 + 2] cycloaddition of enamide with alkyne in the presence of an oxidant [37] , [38] , [39] , [40] , [41] , [42] , [43] , [44] , this iodine-catalyzed formal [4 + 1] cycloaddition of enamide and diazo compound is more practical under overall greener conditions (metal-free, oxidant-free, gram-scale synthesis, no hazardous by-product). This successful construction of pyrroles from enamides greatly highlighted the advantage of this novel iodine-catalyzed radical approach in promoting challenging transformations. Table 5 Synthesis of pyrroles from enamides and diazo compounds Full size table Iodine-catalyzed diazo activation toward olefin epoxidation Since the key iodo-substituted alkyl radical C was well defined by EPR and TEMPO experiment (Fig. 4 ), we wonder if the radical C could be trapped by O 2 to generate peroxide radical J . To our delight, peroxide radical was clearly observed via EPR experiment (see EPR spectra in Supplementary Fig. 5 ). Encouraged by this result, we hypothesized that peroxide radical J would react with olefin to form alkyl radical K , which could undergo fragmentation to generate the epoxide and ethyl 2-oxoacetate along with the regeneration of iodine catalyst (see Supplementary Fig. 6 ). With this in mind, we investigated the reaction of olefin and EDA in the presence of 5 mol% I 2 catalyst in the open air (see details in Supplementary Table 3 ). To our delight, the desired epoxide 7a was obtained in 70% yield, and the yield of 7a was raised to 94% yield under O 2 . No reaction occurred when treating alkene with EDA alone, indicating that I 2 catalyst was crucial for this reaction. Stoichiometric amount of EDA was needed for this reaction, although it was not part of the product 7a . In addition, no desired product 7a was formed at 60 °C, which suggested a plausible activation barrier for this reaction. With this new epoxidation protocol, various alkenes were tested to investigate the scope of the reaction (see Supplementary Table 4 ). Olefin with electron-withdrawing groups (Br, Cl, NO 2 , CO 2 Me, and benzotriazole) worked well, giving the desired epoxide 7a – 7e in good to excellent yields. Olefin with electron-withdrawing groups (OMe and Me) gave messy reactions under the optimal conditions ( 3 f ), owing to the fast decomposition of the products in the presence of iodine. In summary, we report herein a photo-initiated or thermal-initiated iodine-catalyzed diazo activation toward olefin cyclopropanation and epoxidation. An iodo-substituted alkyl radical was identified as the key intermediate experimentally. Significantly, the thermal-initiated and metal-free protocol provided broad substrate scope for cyclopropanation, which was hightlighted by the highly-substituted pyrroles under thermal conditions. Further mechanistic study and synthetic applications of these intriguing iodo-substituted alkyl radicals are currently ongoing in our laboratory. Olefin cyclopropanation under photo-initiated conditions To a 50 mL Schlenk tube with a stir bar was added olefin 2 (0.3 mmol), diazo compound 1 (0.3 mmol) and 3 mL of DCE, then Ru(bpy) 3 Cl 2 ·6H 2 O (2 mg, 0.003 mmol) and I 2 (8 mg, 0.03 mmol) were added. The Schlenk tube was vacuumed and purged with argon three times before it was tightly screw-capped. The reaction mixture was stirred at room temperature under blue light for 24 h. The reaction solution was evaporated, and the residue was purified by column chromatography (PE/EA) to afford the desired product 3a – 3n . Olefin cyclopropanation and pyrrole synthesis under thermal conditions To a 50 mL Schlenk tube with a stir bar was added olefin 2 (0.3 mmol) or enamides (0.3 mmol), diazo compound 1 (0.3 mmol) and 3 mL of DCE, then I 2 (8 mg, 0.03 mmol) were added. The Schlenk tube was vacuumed and purged with argon three times before it was tightly screw-capped. The reaction mixture was stirred at 100 °C for 24 h, and cooled to room temperature. The reaction solution was evaporated, and the residue was purified by column chromatography (PE/EA) to afford the desired product 3a – 3x and 5a – 5t . Olefin epoxidation under thermal-initiated conditions To a 50 mL Schlenk tube with a stir bar was added olefin 2 (0.3 mmol), diazo compound 1 (0.3 mmol) and 3 mL of DCE, then I 2 (4 mg, 0.015 mmol) were added. The Schlenk tube was vacuumed and purged with O 2 three times before it was tightly screw-capped. The reaction mixture was stirred at 80 °C for 2 h, and cooled to room temperature. The reaction solution was evaporated, and the residue was purified by column chromatography (PE/EA) to afford the desired product 7a – 7e . Data availability All data that support the findings of this study are available in the online version of this paper in the accompanying Supplementary Information (including experimental procedures, compound characterization data).